Human-relevant levels of added sugar consumption increase female mortality and lower male fitness in mice Consumption of added sugar has increased over recent decades and is correlated with numerous diseases. Rodent models have elucidated mechanisms of toxicity, but only at concentrations beyond typical human exposure. Here we show that comparatively low levels of added sugar consumption have substantial negative effects on mouse survival, competitive ability, and reproduction. Using Organismal Performance Assays—in which mice fed human-relevant concentrations of added sugar (25% kcal from a mixture of fructose and glucose, modeling high fructose corn syrup) and control mice compete in seminatural enclosures for territories, resources and mates—we demonstrate that fructose/glucose-fed females experience a twofold increase in mortality while fructose/glucose-fed males control 26% fewer territories and produce 25% less offspring. These findings represent the lowest level of sugar consumption shown to adversely affect mammalian health. Clinical defects of fructose/glucose-fed mice were decreased glucose clearance and increased fasting cholesterol. Our data highlight that physiological adversity can exist when clinical disruptions are minor, and suggest that Organismal Performance Assays represent a promising technique for unmasking negative effects of toxicants. Added sugars, those sugars that are added to food during processing or preparation, have increased in the American diet by 50% since the 1970s primarily due to higher consumption of high fructose corn syrup (HFCS) [1] . Over this same period, the proportion of individuals suffering from metabolic diseases has dramatically increased. Excess sugar consumption has been indicated as a factor in the development of cardiovascular disease, fatty liver, metabolic syndrome, obesity and type-2 diabetes [2] , [3] , [4] , [5] , [6] . Mechanisms by which sugar consumption contributes to obesity, de novo lipogenesis, lipid dysregulation and insulin resistance were recently reviewed [7] . Support for these mechanisms is seen in rodent models where high-levels of sugar consumption have been shown to increase adiposity, levels of fasting cholesterol and triglycerides, impair glucose tolerance and to promote chronic inflammation [8] , [9] , [10] , [11] . However, rodent studies evaluating health effects of added sugar have exclusively focused on doses outside the range of human exposure, inviting the criticism that observed adverse effects at high doses might be irrelevant at lower doses currently considered safe. To sensitively assess whether added sugar at human-relevant concentrations decreases mouse health as measured by survival, competitive ability and reproduction (common measures of Darwinian fitness), we utilized Organismal Performance Assays (OPAs). OPAs are sensitive phenotyping approaches that use seminatural conditions to challenge the physiological performance of control and experimental animals in direct competition with each other. It is this competition that reveals performance differences for any measurable component of fitness between treatment and controls. A prototype of the OPA system was first used to detect mating preferences owing to major histocompatibility genes; however, at this time no experimental manipulation occurred and the enclosures only provided an environment in which to make observations [12] . The first experimental comparisons quantified the impact of genetic manipulations, including cousin and sibling-level inbreeding as well as the costs of bearing a selfish genetic element [13] , [14] , [15] ; in all cases, OPAs quantified substantial health impacts in mice that were not detected using standard methodologies. The experimental usage of OPAs in this study marks their début into the realm of environmental exposures and the first time it bears a descriptive title. Here we use OPAs to test if added sugar exposure at a concentration of 25% kcal, a level currently consumed by 13–25% of Americans, decreases mouse health [1] , [16] . To mimic existing sources of added sugar, we selected a diet containing fructose and glucose monosaccharides in a one to one ratio, approximating the 55:42 and 42:53 ratios found in the two common forms of HFCS [17] . Throughout the remainder of the paper, we will refer to the experimental diet as the fructose/glucose (F/G) diet. In addition to OPA measures, we also monitor common metabolic endpoints between experimental and control animals to determine if established toxicity mechanisms correlate with whole organism phenotypes observed in OPAs. Our experiments reveal that moderate F/G feeding has substantial negative effects on mouse survival, competitive ability and reproduction. Specifically, F/G-fed females experienced a twofold increase in mortality, while F/G-fed males controlled 26% fewer territories and produced 25% fewer offspring than controls. Metabolic defects of F/G-fed mice were also detected and included decreased glucose clearance and increased fasting cholesterol. These findings indicate that added sugar consumption at the moderate levels currently consumed by many people have a considerable adverse effect on mammalian health and illustrate that OPAs are a promising technique for unmasking and quantifying the toxicities of various exposures that are of relevance to human health. F/G feeding decreases survival of female mice Survival of females within OPA enclosures was influenced by diet, with F/G-fed females experiencing death rates 1.97 times higher than controls (proportional hazards (PH), P =0.048; Fig. 1a ). There was no difference in survival among replicate populations (PH, P =0.351) nor did the effect of diet differ among replicate populations (PH, P =0.554). 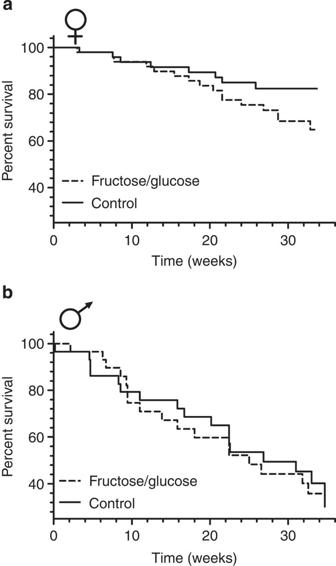Figure 1: Survival of animals within OPA enclosures by sex. (a) Fructose/glucose-fed females experienced a death rate twice that of control females (proportional hazards,n=98,P=0.048). (b) This pattern was not not seen in males (n=58). Figure 1: Survival of animals within OPA enclosures by sex. ( a ) Fructose/glucose-fed females experienced a death rate twice that of control females (proportional hazards, n =98, P =0.048). ( b ) This pattern was not not seen in males ( n =58). Full size image With regards to male survival, no relationship between diet and survival was detected (PH, P =0.777; Fig. 1b ). Survival did not differ among replicate populations (PH, P =0.438) nor did the effect of diet differ among replicate populations (PH, P =0.311). F/G feeding decreases competitive ability of male mice Male competitive ability was adversely affected by F/G feeding, with F/G animals acquiring and defending fewer territories than control males. At week 3 (model intercept), control males occupied 47.9% of total territories and F/G-fed males only occupied 35.5%. This difference was statistically significant (generalized linear mixed model (GLMM), P =0.036). No effects of time or diet by time were detected on territorial acquisition indicating that the competitive advantage of control males was consistently maintained throughout the study. For a complete readout of all mixed model results see Supplementary Table S1 . F/G feeding decreases reproductive success of male mice Female reproductive success was influenced by diet in two distinct and opposing ways ( Fig. 2a ). First, mean reproduction of control females at week 8 (model intercept) was 23.81 with a 95% confidence interval of (21.37, 26.52) offspring per population and for F/G-fed females it was 36.25 (29.98, 43.83) offspring per population. Second, the reproductive output of F/G-fed females decreased over time by −0.0236±0.0057 (mean±s.e.) offspring per week per population relative to controls (GLMM, P <0.0001 (reported slope data are log transformed)). 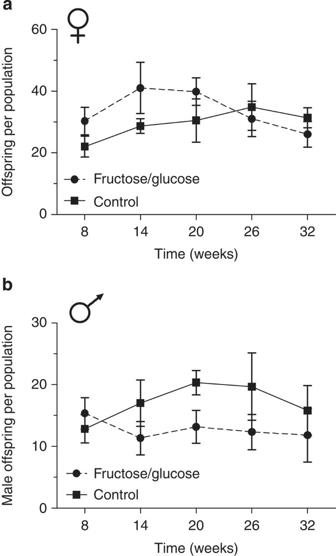Figure 2: Reproduction of animals within OPA enclosures by sex. (a) Fructose/glucose-fed females produced more offspring early in the study, though this effect was negated owing to a decrease in fructose/glucose-fed female reproduction over time (GLMM,P=<0.001). (b) Fructose/glucose-fed males exhibited a 25% reduction in reproductive output due to a decreased rate of reproduction over time relative to controls (GLMM,P=0.034). Reproductive output of both groups was assessed at multiple time points across populations (n=6) for a total of 58 observations. Female reproduction is in terms of total offspring as mitochondrial markers were used. Male reproduction is in terms of male offspring due to using Y-chromosome markers. Lines connect means of the six populations at each time point for each sex (except for week 32, which is based on five populations) and error bars represent s.e. Figure 2: Reproduction of animals within OPA enclosures by sex. ( a ) Fructose/glucose-fed females produced more offspring early in the study, though this effect was negated owing to a decrease in fructose/glucose-fed female reproduction over time (GLMM, P =<0.001). ( b ) Fructose/glucose-fed males exhibited a 25% reduction in reproductive output due to a decreased rate of reproduction over time relative to controls (GLMM, P =0.034). Reproductive output of both groups was assessed at multiple time points across populations ( n =6) for a total of 58 observations. Female reproduction is in terms of total offspring as mitochondrial markers were used. Male reproduction is in terms of male offspring due to using Y-chromosome markers. Lines connect means of the six populations at each time point for each sex (except for week 32, which is based on five populations) and error bars represent s.e. Full size image Male reproductive success was negatively affected by diet, with F/G-fed males siring 25.3% fewer offspring per population than controls ( Fig. 2b ). Differential reproduction was due to a diet by time interaction causing F/G-fed males to sire −0.0175±0.0083 fewer male offspring per week per population than controls (GLMM, P =0.034 (reported slope data are log transformed)). Effect of F/G feeding on body weight and metabolic measures Diet had no effect on the body weight of population founders at week 0 ( Supplementary Fig. S1 ). Nor did the diets have differential impacts on weight over time or between the sexes. Female glucose tolerance, as assessed by intraperitoneal glucose tolerance tests (IPGTT), was influenced by both diet and environment ( Fig. 3a,c ); F/G-fed females had decreased rates of glucose clearance (ANOVA, n =39, P =0.037) as did females in cages before OPA release compared with measures after inhabiting OPA enclosures (ANOVA, n =39, P =0.024). No interaction between diet and environment was detected (ANOVA, n =39, P =0.182). With post-hoc tests, only the difference between dietary groups in cages before OPA entrance was found to be statistically significant. In cages, F/G-fed females had area under the curve values 1.42 times higher than controls (F/G 29,384±2,597: Control 20,719±1,692 mg dl −1 per 120 min (mean±s.e.)). 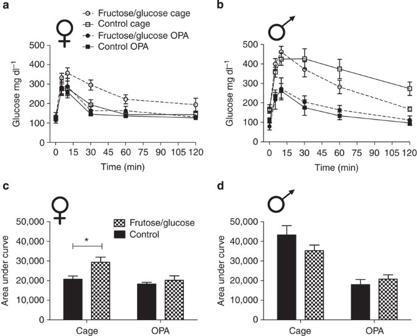Figure 3: Glucose tolerance of animals before and after entrance into OPA enclosures. Both glucose challenge time-course plots (a,b) and integrated area under the curve values are provided (c,d) for both female (a,c) and male (b,d) animals. Fructose/glucose-fed females had reduced glucose tolerance relative to controls (ANOVA,n=24,P=0.037). Animals of both sexes and treatments had reduced glucose clearance in cages before entrance into OPA enclosures (cage) compared with rates after OPA entrance (OPA) (ANOVA F:M,n=24:n=16,P=0.024:P<0.0001). Lines and bars represent means and error bars represent s.e.. *IndicatesP<0.05 with a Bonferroni’s post test. Figure 3: Glucose tolerance of animals before and after entrance into OPA enclosures. Both glucose challenge time-course plots ( a , b ) and integrated area under the curve values are provided ( c , d ) for both female ( a , c ) and male ( b , d ) animals. Fructose/glucose-fed females had reduced glucose tolerance relative to controls (ANOVA, n =24, P =0.037). Animals of both sexes and treatments had reduced glucose clearance in cages before entrance into OPA enclosures (cage) compared with rates after OPA entrance (OPA) (ANOVA F:M, n =24: n =16, P =0.024: P <0.0001). Lines and bars represent means and error bars represent s.e.. *Indicates P <0.05 with a Bonferroni’s post test. Full size image Male glucose clearance rates were not affected by diet (ANOVA, n =25, P =0.519), though, like females, there was a large effect of environment, with males in cages before OPA release having higher levels than post release (ANOVA, n =25, P <0.0001; Fig. 3b,d ). No interaction between diet and environment was detected (ANOVA, n =25, P =0.190). Fasting measures of plasma cholesterol, glucose, insulin and triglycerides of both females and males before OPA entrance were not influenced by diet. All plasma data were also analysed with the sexes combined revealing that total cholesterol was 1.69 times higher in F/G-fed animals ( t -test, t =2.271, df=30, P =0.031; Supplementary Table S2 ). Nearly twice as many F/G-fed females died in OPAs compared with controls and a complex effect of the F/G diet on reproduction was also observed in OPAs. Specifically, F/G females exhibited higher reproductive success early in the study, but a decreasing rate of reproduction as the study progressed. Previous studies demonstrate a positive association between adiposity and reproductive success in females, which is thought to be due to the availability of energy reserves [18] . F/G feeding during the pre-OPA period may have increased adiposity (while not increasing body weight), which could underlie the early elevation in reproductive success. Subsequent reproductive decline and rise in mortality observed in the latter part of the OPA testing could be explained by the mounting physiological insults of the F/G diet interacting with the extreme energetic pressures of simultaneous gestation and lactation, which elevate metabolism by 18–25% [19] . Future studies designed to track these parameters may help in elucidating the relationship between the F/G diet, adiposity, reproductive success and mortality. Overall, F/G-fed males were outcompeted by control animals as measured by competitive ability and reproduction. Though death rates of males were higher than females due to intra-sexual competition, they did not differ between dietary groups. Therefore, it is likely that the lower reproduction of F/G males was due to their decreased ability to defend territories, though other mechanisms may also have decreased reproductive output. Previous work in our system has indicated territorial males sire ≈80% of all pups within an enclosure, as F/G feeding decreased both territorial acquisition and reproduction by ≈25%, it is reasonable to assume that the majority of the reproductive decline is driven by decreased competitive ability, but that a portion of the difference could be due to other reproductive impairments [15] . Previous work demonstrates increased male adiposity due to added sugar at higher exposure levels (for example, Jurgens et al. [8] ); therefore, a plausible explanation is that F/G-fed males could have increased adiposity, despite not having different body weights, leading to a disadvantage in the physical contests required to acquire territories and mates. The sex-specific nature of our OPA findings is interesting though not unprecedented. OPAs revealed a similar mortality pattern, when females harbouring the selfish genetic element known as the t complex experienced an increased risk of mortality while males did not [15] . Likewise, at both cousin and sibling-levels of inbreeding reproductive output in males was impacted to a much higher degree than that of females [13] , [14] . These findings are inline with the notion of a trade-off between reproduction and longevity (for review see Partridge et al. [20] ). Given that the energetic allocation toward offspring is much higher for females than for males it is not surprising that females might incur increased mortality due to a nutritional manipulation, while males would be more likely to decrease reproductive output. The only pre-OPA fasting plasma measure that was associated with the decreased reproduction and increased mortality exhibited by F/G-fed animals was total cholesterol, as no difference was seen in plasma glucose, insulin or triglyceride concentrations. These data suggest that the F/G-fed animals may be suffering from dysregulated lipid metabolism before OPA entrance and supports our hypothesis that differential adiposity may have existed between dietary treatments. In the future, tracking and fractionating cholesterol of animals within OPAs and determining if increased plasma values are predictive of OPA outcomes would be highly informative. Impaired glucose clearance rates of F/G-fed females compared with controls before OPA entrance may reflect a yet to be identified physiological alteration, possibly loss of endocrine capacity, that underlies and predicts increased risk of death within OPA enclosures. However, this impairment in glucose clearance and the underlying physiological alterations that it biomarks is masked within 2 weeks of residing in OPAs, well before the majority of deaths have occurred. Nevertheless, disrupted glucose metabolism throughout the developmental period from weaning into adulthood could cause lasting physiological problems and the glucose disruption may persist in individuals within OPAs, but at levels below the detection limits of current assays. No diet induced differences were seen in regards to male glucose clearance (though both F/G and control-fed males exhibited slower clearance relative to control females) and differential mortality between groups did not occur indicating that perhaps differential glucose clearance is the basis of this sex-specific finding. That both dietary groups, as well as both sexes, markedly increased their rates of glucose clearance after entering OPAs is likely due to increased physical activity permitted by the larger living area as well as the increased energetic demands of reproductive and social activities [21] . As elevated activity leads to increased glucose disposal, metabolic impairments may be masked, making it difficult to establish connections between the pre-OPA alterations in metabolism to the adverse impacts observed in the OPA. The increased rates of mortality and decreased reproduction observed in this study represent the lowest level of added sugar consumption shown to adversely affect mammalian health. These adverse organismal-level findings are detectable while standard clinical measures are either unaltered (body weight, glucose, insulin and triglycerides), or exhibit complicated patterns (cholesterol and glucose tolerance), indicating that the available clinical measures used are not of sufficient sensitivity to reflect the physiological impairments leading to early death in females and reproductive declines in males. With complex organismal-level endpoints like survival, reproduction and competitive ability it is highly unlikely that a single molecular mechanism acting in isolation is responsible for producing the observed phenotype. It is more likely that a variety of mechanisms at the molecular, cellular and higher levels are acting in concert to alter phenotypes. Our glucose clearance and cholesterol results likely represent part of the mechanistic cascade that leads to the decreased survival, reproduction and competitive ability caused by F/G feeding; however, they do not represent its entirety. Clearly more mechanistic work is needed to elucidate the underpinnings of our findings, but current searches into the causes of added sugar-induced diseases are solely focused on extreme exposure levels and therefore may not aid in characterizing effects at human-relevant exposures. The characterization of mechanisms at relevant doses will be more difficult, as high doses are typically used to ‘push the system’ and decrease the amount of time and number of animals required, but the information garnered will be more readily translated to the human condition. Regardless of the mechanisms involved our study characterizes the ultimate impacts of F/G-feeding mice at human-relevant levels. We detected substantial adverse outcomes due to an added sugar exposure consisting of a 1:1 ratio of fructose and glucose amounting to 25% kcal. Our results provide evidence that added sugar consumed at concentrations currently considered safe exerts dramatic adverse impacts on mammalian health [22] , [23] . Many researchers have already made calls for reevaluation of these safe levels of consumption [24] . Although others have advocated for more drastic regulatory measures to curtail sugar consumption [25] . Our study provides experimental data directly supporting mammalian adversity at these ‘safe levels’ and provides a model system in which to investigate the molecular and physiological mechanisms causing this organismal adversity. Though OPAs detected large differences in reproductive output and survival between F/G-fed and control animals, the results from our studies are likely conservative. First, OPAs were terminated at 34 weeks because of the common, diet independent, high rates of male attrition; it is likely that if the study continued for the entirety of the mouse lifespan that reproductive outputs between the treatments would have continued to diverge. Second, at the start of OPA assessment all animals were provided the same sugar enriched diet, because as yet we have no way to keep animals on their respective diets during OPAs. This means that all of the adverse effects of the F/G diet are a consequence of exposure before OPA entrance. Third, our F/G diet was based on a modified chow and not a refined diet, meaning that our F/G-fed animals showed impairment despite having the remainder of their diet being highly nutritive, whole grain-based, with optimum mineral and vitamin composition, analogous to human subjects consuming a healthy diet plus the equivalent of ≈3 cans (354 ml each) of soda per day. By directly assessing the impacts of a treatment on the performance of house mice in OPAs, we are capable of bridging the environmental relevance and longitudinal nature of human studies with the controllability and experimental power of animal models. The data within this paper along with other similar successes using OPAs suggest that this and similar approaches will be an important tool in the detection and quantification of adversity caused by a wide array of treatments [13] , [14] , [15] . Once adversity is detected in OPAs and an adverse phenotype characterized, reductionist techniques can be applied to discover the mechanism and thus provide human translatability. As output measures are similar across experiments, OPAs allow for the direct comparison of disparate treatments. For example, our data indicate that the F/G diet is as detrimental to male reproduction as cousin-level inbreeding ( Supplementary Fig. S2 ). Currently, there is a great need for sensitive toxicity assessment methods that work across a broad range of experimental manipulations. This need is particularly strong for both pharmaceutical science where 73% of drugs that pass preclinical trials fail due to safety concerns and for toxicology, where shockingly few compounds receive critical or long-term toxicity testing [26] , [27] . Likewise, with health-care costs spiralling out of control, partially due to an epidemic of diet-related non-communicable diseases, one could use this approach to identify other dietary components that may link to adverse outcomes (or benefits). Assuredly, the revelation that added sugar consumption at human-relevant concentrations increases death rates and decreases both competitive ability and reproductive output is evidence that OPAs have the potential to identify disease risks that escape notice by standard clinical measures when tested at relevant-human exposures. Animals Wild-derived mice ( Mus musculus ) were used in this study, as laboratory strains do not possess functional behaviours required for OPAs [28] . Individuals were from the 10th and 11th generation of the colony originally described by Meagher et al. [14] . Before release into enclosures animals were housed according to standard protocols under a 12:12 h light:dark cycle with food and water ad libitum . All protocols were approved by and conducted under the animal care guidelines of the University of Utah’s IACUC. Dietary exposure Dietary exposure began at weaning and continued until animals were released into OPAs 26 weeks later. At weaning, litters were split in half and assigned to either the experimental or the control group. The F/G diet (TD.05668; Harlan Teklad, Madison, WI) contained 25% kcal from a 1:1 mixture of fructose and glucose monosaccharides, and has the same ratio of these monosaccharides as sucrose and approximately that of the 55:41 ratio found in HFCS used in beverages (or 42:53 ratio of HFCS used in food preparations) [17] . The control diet (TD.05669; Harlan Teklad, Madison, WI) is identical except for the fructose and glucose is replaced by cornstarch and a small amount of fibre to offset mass differences (see Supplementary Tables S3,S4 ). Upon OPA entrance, all individuals consumed the F/G diet. Though leaving animals on their original diet would be ideal, we have no means to keep animals on their respective diets while they free range. The F/G diet was selected for OPA exposure as we hypothesized that negative effects experienced by the F/G-fed animals during exposure would be maintained/exacerbated. The alternative, feeding the control diet in OPAs, could make differential performance difficult to detect due to potential recovery of individuals pre-exposed to the F/G diet. We gathered intake data on a subset of animals for several weeks starting at weaning and no differential intake was detected. These data are not included for methodological complications owing to using standard metabolic cages designed for laboratory strains with wild-derived mice. Wild type mice escaped readily, nested in feeding areas, jettisoned food and suffered thermoregulatory complications. Furthermore, if differential intake of isocaloric diets occurred during exposure then one would predict that animals on different diets would differ in weight; however, no differential weight was detected. OPA enclosures OPA enclosures are indoors, measure 35 m 2 and are subdivided into six subsections by hardware cloth ( Supplementary Fig. S3 ). Each subsection has food and water that is associated with a set of nest boxes in either one of four ‘optimal’ territories, which contain nest boxes in enclosed structures or two ‘suboptimal’ territories with nest boxes in the open. Optimal nest boxes were made of plastic bins (75 l) with 5 cm diameter entryways and contained four standard mouse cages (also with 5 cm entryways), bedding and food. The suboptimal nest boxes were made of plastic planter boxes fitted with wire lids and 5 cm circular entryways; food containers and one-gallon poultry waterers were adjacent to these boxes and provided ad libitum access. Together, the fences and the two types of boxes created complexity in which mice established nests, territories and hierarchies. OPA enclosures mimic habitat and social environment experienced by mice in nature and population density is representative of wild populations [29] . To assess impacts of added sugar consumption on survival, competitive ability and reproduction six OPA populations were founded by 22–28 individuals, 8–10 males and 14–18 females for a total of 156 individuals (58 male: 98 female). Equal numbers of F/G-fed and control animals were represented for each sex within populations. No male was related at the cousin level or above to other individuals within a given population. Relatedness between females was avoided, though in several populations a single sister-pair was included (a typical condition in nature); when this was the case sister-pairs were balanced across diets. Age of individuals at founding was 29.83±3.60 (mean±s.d.) weeks for males and 30.64±3.60 weeks for females. To prevent breeding before the establishment of male hierarchies, we released placeholder (non-experimental) females with the experimental males at the onset of each population. After 1 week, these females were removed and experimental females released marking week one of the study. Five of six populations lasted 32 weeks, while the other was terminated at 26 weeks due to attrition. A seventh population was established under the same criteria above to collect blood samples from individuals and run for 6 weeks. This population was not used to assess competitive ability, survival or reproduction. Male competitive ability One week before entrance founders were implanted with a unique passive integrated transponder (PIT) tag (TX1400ST, BioMark, Boise ID). A set of PIT antennae and readers (FS2001F-ISO, BioMark, Boise ID) were rotated through populations at regular intervals throughout the study and placed at each feeder. Data were streamed to a computer with logging software (Minimon, Culver City, CA). Dominance was assigned when a male had >75% of the PIT-tag reads at a single location over a multi-day session, and territories were designated as controlled by a F/G or control-fed male-based on the male controlling them. Female data were collected, but not reported here as not enough is known about female dominance to use it to measure performance. Survivorship Founder survivorship was determined by periodic enclosure checks. Dead founders were identified by their PIT-tag or personalized ear punches and removed. Death date was estimated based on three factors: date of last check, the last date an animal was recorded feeding and corpse condition. To avoid disruption of territorial formations and decrease instances of infanticide, which skews reproductive data, researchers entered OPA enclosures only to rotate PIT-tag readers and during pup sweeps (described below). Therefore, corpses were collected at a variety of times since death and in conditions that precluded necropsies. Reproductive success Samples to determine reproductive success of founders were gathered during ‘pup sweeps’ in which pups born during the previous cycle were removed from enclosures, euthanized and had tissue samples taken for genetic analysis. The first sweep occurred during week 8 of the study with additional sweeps every 6 weeks. This schedule prevented offspring born in enclosures from breeding. In five of six populations, five pup sweeps occurred, while in the remaining replicate four were conducted. A total of 1,894 samples were collected with an 315.67±65.54 (mean±s.d.) offspring per population. Population-level reproductive success was determined for F/G and control groups as described previously [14] . In each enclosure male and female founders of each treatment were categorized by a common allelic variant on the Y-chromosome and mitochondrial genome, respectively. Allelic assignments were reversed across populations to avoid possible confounding effects of alleles. We obtained 1,836 (97% of total) mitochondrial and 870 Y-chromosome (92% of total assuming a 1:1 sex ratio) genotypes. This technique decreases the number of microsatellite loci by 10-fold compared with standard parentage analysis, while providing population-level reproductive output for each diet. Metabolic measures Metabolic measures associated with sugar-induced disease were taken including body weight, glucose tolerance, plasma fasting cholesterol, glucose, insulin and triglyceride concentrations. Body weight was assessed in founders at the time of release and each pup sweep, for a total of six time points. Glucose tolerance was assessed in a subset of individuals composed of 24 females (16F/G-fed and 8 controls) and 16 males (8 F/G-fed and 8 controls) at two times, before OPA entrance and again 2 weeks after. Fasting concentrations of plasma cholesterol, glucose, insulin and triglycerides were assessed on a third set of 17 females (8 F/G-fed, 9 control) and 15 males (8 F/G-fed, 7 control) at the end of the dietary exposure. IPGTTs were conducted by giving intraperitoneal injections of 1.5 mg D -glucose per g body weight after an 8-h fast. Blood was collected from the retro-orbital sinus before injection and 5, 10, 30, 60 and 120 min later. Fast duration and bleeding technique were selected because our wild-derived mice do not tolerate fasting or handling like laboratory strains. Blood samples were centrifuged at 10,000 g for 10 min after which 8–10 μl of plasma was decanted and flash frozen. Samples were shipped on dry ice to CHORI and glucose concentrations were assessed by the hexokinase method [30] . Plasma samples for fasting cholesterol, glucose, insulin and triglycerides were collected and shipped in the same manner as those for IPGTT. Plasma glucose was measured as described above. To determine plasma cholesterol and triglyceride concentrations, the infinity triglycerides or cholesterol liquid stable reagent kits (Thermo Scientific, Waltham, MA), were employed according to manufacturer’s instructions. Plasma insulin was measured using a direct sandwich ELISA (Mercodia, Uppsala, Sweden) according to manufacturer’s instructions. The homeostatic model assessment of insulin resistance was calculated by multiplying fasting insulin (mM) and glucose (mM) together, and dividing by 22.5 (ref. 31 ). Statistical analysis Survival was assessed with Cox proportional hazard models, and GLMMs were used for competitive ability and reproduction. A linear mixed model was used to assess body weight, a two-way ANOVA for glucose clearance and either t -tests or Mann–Whitney U- tests for plasma measures. For details see Supplementary Information . How to cite this article: Ruff, J. S. et al. Human-relevant Levels of Added Sugar Consumption Increase Female Mortality and Lower Male Fitness in Mice. Nat. Commun. 4:2245 doi: 10.1038/ncomms3245 (2013).